Plant immunity suppression by an exo-β-1,3-glucanase and an elongation factor 1α of the rice blast fungus Fungal cell walls undergo continual remodeling that generates β-1,3-glucan fragments as products of endo-glycosyl hydrolases (GHs), which can be recognized as pathogen-associated molecular patterns (PAMPs) and trigger plant immune responses. How fungal pathogens suppress those responses is often poorly understood. Here, we study mechanisms underlying the suppression of β-1,3-glucan-triggered plant immunity by the blast fungus Magnaporthe oryzae . We show that an exo-β-1,3-glucanase of the GH17 family, named Ebg1, is important for fungal cell wall integrity and virulence of M. oryzae . Ebg1 can hydrolyze β-1,3-glucan and laminarin into glucose, thus suppressing β-1,3-glucan-triggered plant immunity. However, in addition, Ebg1 seems to act as a PAMP, independent of its hydrolase activity. This Ebg1-induced immunity appears to be dampened by the secretion of an elongation factor 1 alpha protein (EF1α), which interacts and co-localizes with Ebg1 in the apoplast. Future work is needed to understand the mechanisms behind Ebg1-induced immunity and its suppression by EF1α. The cell wall is the outermost layer of fungal cells, composed of diverse polysaccharides interconnected into a three-dimensional structure to shape and protect fungal cells [1] . The fungal cell wall is also dynamic, undergoing remodeling to maintain its integrity, which is required for hyphal growth and development, infection-related morphogenesis and responses to environmental stress [2] . Cell wall remodeling involves fragmentation and re-linkage of polysaccharides by a series of glycosyl hydrolase (GH) family proteins. It has been reported that chitinases Cts1 and Cts2 of the GH18 family in Ustilago maydis [3] , the endo-β-1,3-glucanases ENG1 (GH81), ENG2-5 (GH16) and the β-1,3-glucanosyltransferase Gels (GH72) in Aspergillus fumigatus [4] , [5] , [6] , [7] , play a crucial role in cell wall remodeling. Since the cell wall is the primary contact point of pathogenic fungi with host cells, oligo- and poly-saccharides generated during the cell wall remodeling may leak into the apoplastic region of the fungus-host interface to trigger host immune responses. Oligomers of chitin [8] , [9] , [10] , [11] , [12] and β-1,3-glucans [13] , [14] , [15] , [16] are well-known pathogen-associated molecular patterns (PAMPs) and induce immune responses, both in plant and mammalian cells. For successful infection, fungal pathogens have evolved a battery of mechanisms to prevent elicitation of host defense responses by PAMPs. They may secrete effectors that bind to and prevent these oligosaccharide PAMPs from being recognized by host cells [17] , [18] . Fungal pathogens also secrete GHs and modifying enzymes, which degrade or modify polysaccharides into PAMP-inactive forms. For instance, Verticillium dahliae utilizes the polysaccharide deacetylase PDA1 to deacetylate chitin into chitosan [19] , and fungal pathogens harbor multiple chitinases (GH18) to digest chitin oligomers for evading plant recognition [3] , [20] . Meanwhile, many GH family proteins, including those GH enzymes that degrade plant cell wall polymers to provide nutrients for pathogen invasion [21] , [22] , may also induce plant immunity as PAMPs. One such GH is EIX, a GH11 protein in Trichoderma viride implicated in xylan degradation and the first characterized PAMP in plants [23] , [24] . However, it remains largely unknown how fungal pathogens mask these GH proteins to prevent them from causing plant immune responses. Magnaporthe oryzae is the causative agent of rice blast disease, one of the most destructive crop diseases worldwide [25] . In the cell wall of M. oryzae , chitin and β-1,3-glucan are the two major forms of polysaccharide [2] . To suppress chitin-triggered immunity, the pathogen specifically expresses and secretes the chitin-binding effector Slp1 [14] , [17] and a chitinase MoChia1 (GH18) involved in hydrolyzing oligo-chitins into monomeric GlcNAc, during infection [26] , [27] . Furthermore, M. oryzae synthesizes and accumulates α-1,3-glucan on the surface of the cell wall to sequester β-1,3-glucan from plant recognition [28] . In addition, M. oryzae expresses several β-1,3-glucanosyltransferases (GH72) that are important for cell wall remodeling and virulence [29] . However, the M. oryzae genome encodes a much larger repertoire of GHs that have not been functionally characterized [30] , [31] , including seven GH17 family members similar to Scw4p, Scw10p, Scw11p, and Bgl2p, which act as endo-β-1,3-glucanases during cell wall remodeling in Saccharomyces cerevisiae [32] , [33] , [34] . This study set out to investigate how M. oryzae safeguards cell wall remodeling involving β-1,3-glucan modification during infection. We identified a fungal-conserved exo-β-1,3-glucanase of the GH17 family, named Ebg1, which is vital for cell wall integrity and virulence of M. oryzae . Ebg1 degrades β-1,3-glucan into glucose to avoid β-1,3-glucan-triggered plant immunity. However, Ebg1 itself is also a PAMP. Interestingly, M. oryzae possesses a EF1α protein which interacts and co-localizes with Ebg1 in the apoplastic space to prevent it from triggering host immune responses. Magnaporthe oryzae gene EBG1 is required for cell wall remodeling and pathogenicity The M. oryzae genome contains seven GH17 genes encoding putative β-1,3-glucanases: MGG_04582 , MGG_00863 , MGG_10591 , MGG_09619 , MGG_04689 , MGG_06023 , and MGG_10400 [30] , [31] (Supplementary Fig. 1 ). To investigate their roles in cell wall remodeling and plant infection, we generated targeted gene deletion mutants for each of these genes, including MGG_04582 named as EBG1 , which shows similarity at its C-terminus to the S . cerevisiae Scw11p of GH17 involved in cell wall integrity [34] (Supplementary Fig. 1 ). Bioassays showed that the two deletion mutants of EBG1 (Supplementary Fig. 2a , b ) are similar to the wild-type strain P131 in mycelial growth, conidiation, conidial germination and appressorium formation (Supplementary Fig. 2c – h ). However, as shown in Fig. 1a, b , ∆ ebg1 mutants are highly sensitive to cell wall perturbing reagents such as calcofluor white (CFW) and congo red (CR). When grown on complete medium supplemented with CFW or CR, mycelial growth of P131 was reduced by 25.8% and 10.9%, respectively, whereas growth of ∆ ebg1 mutants was reduced by 41.5% and 14.3%, respectively. RT-qPCR analysis indicated that MGG_04582 is constitutively expressed in vegetative hyphae, and exhibited differential expression during plant infection and invasive growth (Fig. 1c ). When considered together, these observations indicate that MGG_04582 is involved in cell wall remodeling during hyphal growth and plant infection. Fig. 1: Magnaporthe oryzae EBG1 is important for the cell wall integrity, virulence, invasive growth, and suppressing host ROS. a , b Δ ebg1 mutants display defects in cell wall integrity. The wild-type P131, the EBG1 deletion mutant Δ ebg1 and a complemented transformant Δ ebg1 / EBG1 were cultured on the complete medium (CM) plates supplemented with 200 μg/ml CR or 100 μg/ml CFW at 28°C for 5 days ( a ), and their growth inhibition rates were calculated in ( b ). CR, Congo Red; CFW, Calcofluor white. c Relative expression levels of EBG1 in vegetative hyphae (HY) and at different infection stages. RNAs were extracted from inoculated barley leaves at indicated hours post inoculation (hpi) and vegetative hyphae. Relative expression of EBG1 referred to MoActin was calculated and the value at 0 hpi was set as 1. d , e Δ ebg1 mutants show significantly reduced virulence on both rice and barley leaves. Detached leaves were sprayed with conidia suspensions (5 × 10 4 spores/ml) of P131, Δ ebg1, and Δ ebg1 / EBG1 strains, and photographed at 5-day post inoculation (dpi) ( d ). Typical lesions and dark brown spots formed on rice and barley leaves were counted per leave ( e ). f – i Δ ebg1 mutants are reduced in invasive growth. Rice sheath were inoculated with conidia suspensions of P131, Δ ebg1 , and Δ ebg1 / EBG1 strains. The hyphal growth was observed and photographed at 18, 36, and 48 hpi with a Nikon 90i microscope ( f ). Scale bars = 20 μm. Δ ebg1 mutants are reduced in appressorial penetration rates, which were calculated at 18 and 30 hpi ( g ). The percentage of distinct types of infection hyphae, e.g. one branch, two branches, and three or more branches, were examined at 36 hpi ( h ). IH, infection hyphae. The percentages of cell-to-cell movement of infection hyphae were calculated at 48 hpi ( i ). j , k Δ ebg1 mutants induce ROS production in infected rice sheath cells. Rice sheath cells inoculated with the conidia suspensions (1 × 10 5 spores/ml) of P131, Δ ebg1 , and Δ ebg1 / EBG1 strains were stained with DAB at 30 hpi ( i ). Scale bars = 20 μm. The percentages of DAB-stained cells versus infected cells were calculated ( j ). l , m Diphenyleneiodonium (DPI), an inhibitor of NADPH oxidase, can partially restore the invasive growth of Δ ebg1 mutant. Inoculated rice sheath cells were treated at 12 h post inoculation with 0.5 μM DPI dissolved in 1% DMSO and with 1% DMSO as a mock treatment. The growth of infection hyphae was observed and photographed at 36 hpi using a Nikon 90i microscope( l ). Scale bars = 20 μm. Meanwhile, infection sites with distinct types of infection hyphae, e.g. one branch, two branches, and three or more branches, were scored to calculate their percentages ( m ). IH, infection hyphae. For all the above statistics, error bars denote standard deviations from three biological replicates. ** and * indicate p < 0.01 and p < 0.05 significant differences compared with the corresponding WT controls. One-way ANOVA with post-hoc Turkey tests were used in ( b ), ( c ), ( e ), ( g – i ) and ( k ), and two-tailed Student’s t-test were used in ( m ). Source data with statistic analysis are provided in a Source data file. Full size image We next assayed the effect of deletion of EBG1 on fungal pathogenicity. Following spray inoculation of conidia on rice and barley leaves, the wild-type and ∆ ebg1/EBG1 complementation strains generated typical spreading blast lesions mixed with some smaller dark brown flecks, whereas the ∆ ebg1 mutant mainly formed tiny dark brown flecks mixed with very few typical spreading blast lesions (Fig. 1d, e ), indicating that EBG1 is important for virulence. In addition, the total number of lesions formed by the ∆ ebg 1 mutant was significantly less than those formed by the isogenic wild-type and complementation strains (Fig. 1d, e ), suggesting that EBG1 may also be involved in the initial infection of host cells. EBG1 is important for invasive hyphae growth and suppression of host ROS during rice blast infection To understand how EBG1 is involved in virulence, we compared the infection process of the wild-type P131, the ∆ ebg1 mutant, and ∆ ebg1/EBG1 complementation strains in rice leaf sheaths and barley leaves. As shown in Fig. 1f–h , at 18-h post-inoculation (hpi), over 76% of appressoria formed by the wild-type and ∆ ebg1/EBG1 complementation strains penetrated rice leaf sheath cells and developed primary infection hyphae (IH), while only 33% of ∆ ebg1 mutant appressoria penetrated rice cells. At 30 hpi, the appressorium penetration rate of P131 and ∆ ebg1/EBG1 reached 93%, but only 70% for the ∆ ebg1 mutant. Furthermore, at 36 hpi, more than 58% of IH of P131 and ∆ ebg1/EBG1 formed multiple branches in primary invaded rice cells, whereas only 33% of IH of ∆ ebg1 formed multiple branches, indicating that development of ∆ ebg1 IH inside plant cells is attenuated. In addition, at 48 hpi, IH of P131 and ∆ ebg1/EBG1 at more than 75% sites expanded into adjacent rice cells, while only 30% of IH of ∆ ebg1 proliferated into adjacent cells (Fig. 1f, i ). The infection process of the three strains in barley leaf cells was similar to that observed in rice leaf sheath cells (Supplementary Fig. 3a–c ). Taken together, we conclude that EBG1 is important for efficient appressorium-mediated penetration and invasive hyphal growth. We observed that ∆ ebg1 predominantly formed tiny dark brown flecks following plant infection (Fig. 1d, e ) and we therefore, wondered whether EBG1 plays a role in suppressing host immune responses, such as the generation of reactive oxygen species (ROS). We, therefore examined ROS accumulation in both rice leaf sheath cells and barley leaf epidermal cells infected by P131, ∆ ebg1 , and ∆ ebg1/EBG1 strains using 3,3′-diaminobenzidine (DAB), a dye that detects hydrogen peroxide (H 2 O 2 ). Strong ROS accumulation was detected in rice cells surrounding 70% of infection sites of Δ ebg1 as opposed to about 15% of P131 and Δ ebg1/EBG1 (Fig. 1j, k ). Similar ROS accumulation was observed in the barley cells infected by the three strains (Supplementary Fig. 3d, e ), indicating that EBG1 is required to suppress the host ROS burst during plant infection. To determine whether ROS accumulation is a key factor in reducing the virulence of Δ ebg1 , we tested whether invasive growth of the mutant could be remediated by addition of diphenyleneiodonium (DPI), an inhibitor of flavoenzymes including NADPH oxidase, a key enzyme for ROS generation. DPI treatment rescued the multi-branching phenotype of IH at 45% infection sites formed by Δ ebg1 at 36 hpi on rice leaf sheath cells, which was significantly higher than the control experiment (21.7%) carried out with DMSO, which was used as DPI solvent (Fig. 1l, m ). The suppression of ROS generation was therefore able to restore impaired IH growth of Δ ebg1 mutants, albeit not to the level of P131 (58.3%) or the complemented Δ ebg1/EBG1 strain (56.7%). Similarly, DPI treatment partially rescued the invasive growth of Δ ebg1 in barley epidermal cells (Supplementary Fig. 3f , g ). Therefore, host ROS accumulation is an important factor but not the only reason for impaired biotrophic growth of Δ ebg1 mutants. M. oryzae Ebg1 is a secreted protein To determine the subcellular localization of Ebg1 protein, we generated an EBG1 - GFP construct and expressed it in a Δ ebg1 mutant. Fifteen transformants were obtained, and all recovered wild-type mycelial growth on CM medium supplemented with CFW or CR (Supplementary Fig. 4a ), indicating that Ebg1-GFP is a functional chimeric protein. Using one of these transformants, we then investigated the subcellular distribution of the Ebg1-GFP signal in vegetative hyphae, conidia, appressoria, and infection hyphae. In vegetative hyphal cells, the fluorescent signals were present at the hyphal tip, septa, and around the cell wall whereas signals were also unevenly aggregated in conidia, germinated conidia and appressoria, most likely in the endoplasmic reticulum (Supplementary Fig. 4b ). In infection hyphae, Ebg1-GFP signals were mainly distributed around the cell wall (Fig. 2a ) and showed a distinct pattern of localization compared to the cytoplasmic effector Pwl2. We generated a strain expressing Ebg1-GFP and Pwl2-mCherry and infected rice seedlings. At 26 hpi, Pwl2-mCherry was observed in the biotrophic interfacial complex (BIC), whereas Ebg1-GFP was present in the cell wall of invasive hyphae. A similar pattern of localization of Ebg1-GFP was observed at 40 hpi, with Pwl2-mCherry localizing at nascent BICs in newly invaded cells (Fig. 2b, c ). These results suggested that Ebg1 is likely a secreted cell wall and apoplastic protein. To test this idea, we measured Ebg1 in the filtrate and mycelium of liquid CM cultures using immunoblot analysis. As shown in Fig. 2d , two main Ebg1-GFP bands were detected in culture filtrates as well as in mycelium by an anti-GFP antibody, one of which was the molecular weight as expected for the full-length Ebg1-GFP fused protein, and the other was likely a processed form of the Ebg1-GFP. We also validated the activity of the Ebg1 signal peptide (SP) sequence predicted by SignalP using a yeast secretion assay. We observed that the EBG1 full-length sequence ( EBG1-FL ) but not the SP-deleted sequence ( EBG1-∆ SP) fused to SUC2 was able to deliver invertase into the growth medium with raffinose, as shown in Fig. 2e . When considered together, these data indicate that Ebg1 is a secreted protein. Fig. 2: Ebg1 is a secreted protein. a Subcellular localization of Ebg1-GFP in the infection hyphae of M. oryzae . The Ebg1-GFP fluorescence from the Δ ebg1 / EBG1 complemented transformants was distributed mainly around the cell wall and the tip of infection hyphae. Images were captured at 48 h post inoculation (hpi) on barley epidermal leaves. Scale bars = 20 μm. b , c Laser confocal micrographs of M. oryzae strain expressing Ebg1-GFP and Pwl2-mCherry. The Ebg1-GFP/Pwl2-mCherry image shows the overlay of the GFP channel and mCherry channel. A merged image shows the overlay of GFP channel, mCherry channel, and the brightfield channel. Images were captured at 26 hpi ( b ) and 40 hpi ( c ) on rice cultivar LTH. Scale bars = 10 μm. d The Ebg1 protein was detected both in vegetative hyphae and cultured medium. A Δ ebg1 / EBG1 complemented transformant and a P131/ GFP transformant were cultured in liquid CM, and total proteins extracted from the mycelia and from the culture filtrates were immunoblotted with an anti-GFP antibody. Intact and truncated versions of Ebg1-GFP were labeled with a black solid triangle and an open triangle, respectively. Anti-actin antibody were used to confirm the protein samples of vegetative hyphae. e Ebg1 has a functional signal peptide directing its secretion. The EBG1 full-length sequence ( EBG1-FL ) and signal peptide deleted sequence ( EBG1- ΔSP) were constructed into the pSUC2 vector and transformed into yeast YTK12(SUC2-) for the invertase secretion test. The yeast transformants with EBG1-FL grew well on the YPRAA medium containing raffinose and antimycin A, whereas EBG1- Δ SP failed to grow on the same medium. Yeast strains with Avr1b and Mg87 were used as positive and negative controls, respectively. Full size image Ebg1 is an exo-β-1,3-glucanase important for the evasion of plant basal immunity Since the three well-known GH17 family proteins, Bgl2p, Scw4p, and Scw10p from S. cerevisiae exhibit endo-glucanase activity [32] , [33] , [34] , we wondered whether the M. oryzae Ebg1 also functions as a glucanase. We first tested the growth of P131 and the Δebg1 mutant on minimal medium with different carbohydrates as sole carbon sources (Fig. 3a ). Vegetative growth of P131 and Δ ebg1/EBG1 was comparable on plates supplied with glucose, laminarin, cellulose, and chitin (Fig. 3a, b ). However, the colony diameter of the Δ ebg1 mutant was much smaller on minimal medium supplemented with laminarin, compared with that of Δ ebg1 on other carbohydrate substrates (Fig. 3a, b ). These results suggested that Ebg1 is a putative glucanase that can act on laminarin, a carbohydrate composed of β-1,3-glucan and β-1,6-linked branches. Fig. 3: M. oryzae Ebg1 is an exo-β-1,3-glucanase. a , b The growth of the Δ ebg1 mutant on minimal medium with laminarin is significantly reduced compared to that on minimal medium with other polysaccharides as sole carbon sources. P131, Δ ebg1 mutant, and Δ ebg1 / EBG1 were cultured on minimal medium supplemented with 1% (w/v) glucose, laminarin, cellulose, or chitin at 28 °C for 5 days, photographed ( a ) and measured for colony diameter ( b ). Laminarin, water-soluble β-1,3-linked glucans with occasional β-1,6-linked branches; Cellulose, β-1,4-linked glucans; Chitin, β-1,4-linked N-acetylglucosamine polymers. Error bars denote standard deviations from three biological replicates. ** p < 0.01 using Student’s t test. Source data with statistic analysis are provided in a Source Data file. c Purification of Ebg1-6His protein from the CM culture filtrates of M. oryzae . The crude proteins from liquid CM culture filtrates of an EBG1-6His strain were purified with ion-exchange chromatography and polyhistidine binding resin before subjected to SDS–PAGE analysis with CBB staining (left panel) and immunoblot analysis using the anti-His antibody (right panel). Lanes 1 and 3: 10 μg of crude proteins; lanes 2 and 4: 0.5 μg and 0.25 μg of purified Ebg1-6His protein. The black solid triangles indicate the correct size for intact Ebg1-6His protein at around 55 kDa, and the open triangle indicates the truncated protein. d Purified Ebg1-6His protein hydrolyzed laminarins into glucose. Left panel: laminarioligosaccharides with different lengths (L2–L6) and glucose were loaded on HPLC as standard substances. Middle panel: untreated laminarin were loaded as blank control, and glucose was barely detected. Right panel: laminarin treated with purified Ebg1-6His protein were loaded for HPLC analysis and only glucose was detected from the reaction. Glc, glucose; L2, Laminaribiose; L3, Laminaritriose; L4, Laminaritetraose; L5, Laminaripentaose; L6, Laminarihexaose. e Purified Ebg1-6His protein hydrolyzed β-1,3-glucan, laminarin, and laminarioligosaccharides, but neither cellulose nor chitin. The hydrolytic activities of Ebg1-6His on different polysaccharides or oligosaccharides were assayed by detecting the amount of released glucose. Boiled Ebg1-6His protein lost its hydrolytic activity on laminarin. Error bars denote standard deviation. f ROS burst was triggered by β-1,3-glucan but not glucose in rice. Leaf disks of 4-week-old rice plants were incubated with 20 μg/ml β-1,3-glucan or glucose, and the luminol-based ROS burst was detected for 60 min constantly. RLU, relative light units. Error bars denote standard deviation, n = 8. g MAPK activation was triggered in rice leaves by β-1,3-glucan but not glucose. Two-week-old rice seedlings were incubated with 40 μg/ml β-1,3-glucan or glucose for indicated time. Activated MAPKs were detected by immunoblotting with the phospho-p42/44 MAPK antibody. The anti-actin blot was used as a loading control. The experiment was repeated three times with similar results. Full size image To biochemically characterize Ebg1, an EBG1-6His construct driven by the constitutive RP27 promoter was transformed into the Δ ebg1 mutant. The expressed Ebg1-6His protein was concentrated and affinity-purified from culture filtrates, and validated by SDS–PAGE with coomassie blue staining and immunoblot analysis (Fig. 3c ). The purified Ebg1-6His protein was then incubated with laminarin, and hydrolytic products examined by HPLC. As shown in Fig. 3d , glucose was detected as the sole product. Furthermore, when laminarin oligosaccharides of different lengths, e.g., L2, L3, L4, L5, and L6, were incubated with Ebg1-6His, glucose was also the sole hydrolytic product observed (Supplementary Fig. 5a ). Therefore, in follow-up tests, the amount of glucose released into the solution was measured to estimate the hydrolytic activity of Ebg1-6His on various polysaccharides. Ebg1-6His showed strong hydrolysis activity on soluble laminarin and laminarin oligosaccharides, with slightly weaker activity on insoluble β-1,3-glucan, but no activity on cellulose and chitin, both of which are β-1,4-linked polymers (Fig. 3e ). In addition, we observed that Ebg1-6His lost its hydrolase activity after boiling (Fig. 3e ). The optimal pH and temperature of Ebg1-6His were pH 5.0 and 50 °C, respectively (Supplementary Fig. 5b, c ). It has been reported that β-glucan from pathogenic fungi induces PAMP-triggered immunity [13] , [14] . Since Ebg1 appears to be an exo-β-1,3-glucanase that can release glucose from β-1,3-glucans, this prompted us to investigate whether Ebg1 might protect M. oryzae from β-1,3-glucan-mediated triggering plant immune responses. To test this hypothesis, we measured the ability of β-1,3-glucan to induce plant immunity. We found that β-1,3-glucan, but not glucose, is capable of inducing a ROS burst and MAPK activation in rice leaves, as shown in Fig. 3f, g . Previous studies showed that GH17 family members have two conserved glutamic acid residues [35] , and Ebg1 has these residues at positions 378 and 476 (Supplementary Fig. 6a ). To determine whether the two residues are important for Ebg1 activity, we generated an EBG1 construct in which the two residues were simultaneously replaced by glutamine, named EBG1 E378Q/E476Q , and transformed this into the Δ ebg1 mutant (Supplementary Fig. 6a ). Fifteen transformants were obtained, and all of them, including Δ ebg1/EBG1 E378Q/E476Q -1 and -6, were similar to Δ ebg1 in phenotype, exhibiting defects in the utilization of polysaccharides with β-1,3 glycosidic linkage (Supplementary Fig. 6b , c ), sensitivity to CFW and CR (Supplementary Fig. 6d , e ), and a significant reduction in virulence (Supplementary Fig. 6f , g ). We then tested the exo-β-1,3-glucanase activity of purified Ebg1 E378Q/E476Q -6His protein and found that the mutant protein largely lost enzymatic activity (Supplementary Fig. 6h , i ). Taken together, these results provide evidence that EBG1 E378Q/E476Q is unable to rescue the defects of Δ ebg1 mutants, indicating that Glu-378 and Glu-476 are required for Ebg1 to act as a functional exo-β-1,3-glucanase, which is important for its role in virulence of M. oryzae . Additionally, exogenous application of purified protein Ebg1-6His could rescue the infection defect of Δ ebg1 strain (Supplementary Fig. 7a – d ) and suppress the host ROS accumulation triggered by Δ ebg1 infection (Supplementary Fig. 7e – h ), further confirming that Ebg1 plays an important role in suppressing plant basal immunity. Ebg1 can act as a PAMP, independent of its enzymatic activity Many GH family proteins are known to act as PAMPs, including the GH12 family protein PsXEG1 from P. sojae [36] and the GH18 family protein MoChia1 from M. oryzae [26] . Therefore, we reasoned that Ebg1 might also be recognized as a PAMP. Ebg1 contains an N-terminal signal peptide (SP, 1-21aa) and a GH17 domain at the C-terminal region (269-526aa) (Fig. 4a ). When full-length EBG1 was transiently expressed through Agroinfiltration in N. benthamiana , it caused conspicuous cell death (Fig. 4b ). Since Ebg1 is expressed in both full-length and truncated forms (Figs. 2 d and 3c ), we tested whether the individual N- and C-terminal truncated Ebg1 proteins can induce cell death. When transiently expressing each truncated protein carrying the signal peptide with either the N-terminus (Ebg1-N, 1-267aa) or C-terminal part of Ebg1 (Ebg1-C, signal peptide 1-21aa fused in-frame to 268-541aa), both the N- and C-terminal truncated proteins induced cell death responses in tobacco leaves (Fig. 4a, b ). In addition, the Ebg1 E378Q/E476Q mutant also induced cell death responses in tobacco leaves. However, Ebg1 or Ebg1 E378Q/E476Q protein without the signal peptide ( EBG1-Δsp and EBG1 E378Q/E476Q -Δ sp) failed to trigger a response (Fig. 4a, b ). Immunoblotting confirmed that full-length Ebg1, and each mutant or truncated protein were all expressed as expected (Supplementary Fig. 8a ). These results provide evidence that Ebg1 can trigger cell death in tobacco leaves independent of its enzymatic activity. Fig. 4: Ebg1 elicits tobacco cell death and activates rice immune responses. a Schematic diagram of M. oryzae Ebg1 protein. The signal peptide is indicated in orange, and the GH17 hydrolase domain is indicated in blue. Ebg1, Full-length protein; Ebg1-N, the N-terminal half of Ebg1 (1-267aa); Ebg1-C, the signal peptide linked with the C-terminal half of Ebg1 (1-21aa fused to 268-541aa). Ebg1-Δsp, Ebg1 protein without the signal peptide. b Ebg1 induced cell death in N. benthamiana . Tobacco leaves infiltrated with Agrobacterium strains carrying BAX , EBG1 , EBG1-N , EBG1-C , EBG1-Δ sp, EBG1 E378Q/E476Q , and EBG1 E378Q/E476Q -Δsp were photographed at 5-day post infiltration (dpi) and stained with trypan blue. The numbers indicate leaves with cell death versus total treated leaves. EV, empty vector was used as a negative control, and BAX was used as a positive control. c Cell death triggered by Ebg1 in N. benthamiana requires NbBAK1 . Tobacco plants were subjected to VIGS by inoculation with TRV: GFP or TRV: NbBAK1 . Three weeks after VIGS treatment, GFP , INF1 , and EBG1 were transiently expressed in the gene-silenced leaves and then leaves were photographed at 7 dpi. The numbers indicate leaves with cell death versus total treated leaves. d Purified Ebg1 protein induced ROS spiking in rice cultivar ZH11. Leaf disks of 4-week-old rice plants were incubated with 80 μg/ml Ebg1-6His or Ebg1 E378Q/E476Q -6His, and the luminol-based ROS burst was detected for 35 min constantly. Ef1a-6His protein and mock treatment were used as negative controls. RLU, relative light units. Error bars denote standard deviation, n = 8. e Purified Ebg1 protein induced ROS generation in rice cultivar Kitaake and reduced ROS level in two OsSerk2 RNAi lines. Leaf disks of 4-week-old rice plants were incubated with 80 μg/ml Ebg1-6His, and the luminol-based ROS burst was detected for 35 min constantly. Mock treatment was used as the negative control. RLU, relative light units. Error bars denote standard deviation, n = 6. Full size image To investigate the basis of cell death observed in the N. benthamiana assays, we decided to test the role of BAK1, a key protein kinase in multiple PAMP pathways, which directly interacts with different PAMP receptors [37] . To test the potential role of BAK1 in cell death induced by Ebg1, we silenced the BAK1 gene of N. benthamiana using a tobacco rattle virus (TRV)-based virus-induced gene silencing (VIGS) system before expressing EBG1 or INF1 by agroinfiltration [38] . INF1 failed to trigger cell death in BAK1 -silenced plants (Fig. 4c ), consistent with a previous report that BAK1 is required for INF1-induced cell death [37] . Interestingly, Ebg1 was also unable to induce a cell death response in BAK1 -silenced plants (Fig. 4c ). For these experiments, we confirmed that both INF1 and Ebg1 were expressed at the expected size in plants transformed with TRV: NbBAK1 or TRV: GFP by immunoblots (Supplementary Fig. 8b ) and that BAK1 expression was significantly reduced in the TRV: NbBAK1 -transformed plants compared to the TRV: GFP -transformed plants, as revealed by RT-qPCR analysis (Supplementary Fig. 8c ). We conclude that BAK1 is required for Ebg1-triggered cell death in N. benthamiana . Using Ebg1-6His protein purified as described above, we further tested whether Ebg1 can induce rice PAMP responses, such as ROS generation and MAPK activation [39] . When rice leaf disks were supplemented with purified Ebg1-6His and Ebg1 E378Q/E476Q -6His, ROS generation and MAPK activation were clearly observed (Fig. 4d and Supplementary Fig. 8d ), confirming that the elicitor activity of Ebg1 in rice plants is independent of its enzymatic activity. The rice genome contains two BAK1 homologs OsSerk1 and OsSerk2 , which are key regulators in rice development and immunity [40] , [41] , [42] . We also observed that the Ebg1-6His-induced ROS burst was impaired in RNAi rice lines of OsSerk2 as compared to the wild type cultivar (Fig. 4e ), suggesting that OsSerk2 contributes to the Ebg1-induced rice immunity responses. Ebg1 interacts with translation elongation factor 1 alpha protein to evade plant immunity To investigate how M. oryzae evades Ebg1-triggered host innate immunity during infection, we searched for proteins that interact with Ebg1 by yeast two-hybrid analysis (Y2H). 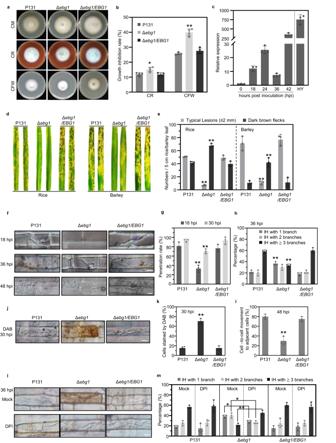Fig. 1:Magnaporthe oryzae EBG1is important for the cell wall integrity, virulence, invasive growth, and suppressing host ROS. a,bΔebg1mutants display defects in cell wall integrity. The wild-type P131, theEBG1deletion mutant Δebg1and a complemented transformant Δebg1/EBG1were cultured on the complete medium (CM) plates supplemented with 200 μg/ml CR or 100 μg/ml CFW at 28°C for 5 days (a), and their growth inhibition rates were calculated in (b). CR, Congo Red; CFW, Calcofluor white.cRelative expression levels ofEBG1in vegetative hyphae (HY) and at different infection stages. RNAs were extracted from inoculated barley leaves at indicated hours post inoculation (hpi) and vegetative hyphae. Relative expression ofEBG1referred toMoActinwas calculated and the value at 0 hpi was set as 1.d,eΔebg1mutants show significantly reduced virulence on both rice and barley leaves. Detached leaves were sprayed with conidia suspensions (5 × 104spores/ml) of P131, Δebg1,and Δebg1/EBG1strains, and photographed at 5-day post inoculation (dpi) (d). Typical lesions and dark brown spots formed on rice and barley leaves were counted per leave (e).f–iΔebg1mutants are reduced in invasive growth. Rice sheath were inoculated with conidia suspensions of P131, Δebg1, and Δebg1/EBG1strains. The hyphal growth was observed and photographed at 18, 36, and 48 hpi with a Nikon 90i microscope (f). Scale bars = 20 μm. Δebg1mutants are reduced in appressorial penetration rates, which were calculated at 18 and 30 hpi (g). The percentage of distinct types of infection hyphae, e.g. one branch, two branches, and three or more branches, were examined at 36 hpi (h). IH, infection hyphae. The percentages of cell-to-cell movement of infection hyphae were calculated at 48 hpi (i).j,kΔebg1mutants induce ROS production in infected rice sheath cells. Rice sheath cells inoculated with the conidia suspensions (1 × 105spores/ml) of P131, Δebg1, and Δebg1/EBG1strains were stained with DAB at 30 hpi (i). Scale bars = 20 μm. The percentages of DAB-stained cells versus infected cells were calculated (j).l,mDiphenyleneiodonium (DPI), an inhibitor of NADPH oxidase, can partially restore the invasive growth of Δebg1mutant. Inoculated rice sheath cells were treated at 12 h post inoculation with 0.5 μM DPI dissolved in 1% DMSO and with 1% DMSO as a mock treatment. The growth of infection hyphae was observed and photographed at 36 hpi using a Nikon 90i microscope(l). Scale bars = 20 μm. Meanwhile, infection sites with distinct types of infection hyphae, e.g. one branch, two branches, and three or more branches, were scored to calculate their percentages (m). IH, infection hyphae. For all the above statistics, error bars denote standard deviations from three biological replicates. ** and * indicatep< 0.01 andp< 0.05 significant differences compared with the corresponding WT controls. One-way ANOVA with post-hoc Turkey tests were used in (b), (c), (e), (g–i) and (k), and two-tailed Student’s t-test were used in (m). Source data with statistic analysis are provided in a Source data file. Using signal peptide-deleted coding sequence of EBG1 ( EBG1-∆ SP) as the bait, we obtained nine putative Ebg1-interacting proteins from a cDNA library constructed with M. oryzae -infected rice leaves (Supplementary Table 1 ). Interestingly, among the Ebg1-interacting proteins was an elongation factor 1 alpha (EF1α) encoded by MGG_03641 , which contains three EF-Tu domains: domain 1 for GTP binding, domains 2 and 3 with beta-barrel structures (Fig. 5a ). Ebg1 was confirmed to interact with EF1α but not with the other two closely related EF-Tu domain-containing proteins, MGG_08162 and MGG_02504, by the Y2H assay (Supplementary Figs. 9 , 10a, b ). In addition, EF1α interacts with Ebg1 and the loss-of-enzyme activity mutant Ebg1 E378Q/E476Q via its domain 2 and domain 3 in a Y2H assay (Fig. 5b ). Fig. 5: M. oryzae EF1α interacts with Ebg1 and prevent plant immune responses triggered by Ebg1. a Schematic diagram of M. oryzae EF1α protein. Domain 1 with putative GTP binding activity, Domain 2 and Domain 3 with beta-barrel structure, are indicated in green, gray, and orange boxes, respectively. EF1α-D1, EF1α-D2, EF1α-D3 are truncations of EF1α protein with indicated domains. b The yeast two-hybrid assays showing that EF1α-D2 and EF1α-D3, but not EF1α-D1 interact with Ebg1, Ebg1 E378Q/E476Q , Ebg1-N, and Ebg1-C. c Co-immunoprecipitation assays showing that EF1α interacts with Ebg1 in the extracellular matrix of M. oryzae . The EBG1-GFP and EF1α-3Flag vectors were co-transformed into M. oryzae P131 for Co-immunoprecipitation assay. Total proteins from liquid CM culture filtrates of the transformant were subjected to GFP or Flag pull-down analysis. Total proteins or Co-IP elutions were detected by anti-GFP antibody or anti-Flag antibody. The P131 strain expressing SLP1-GFP and EF1α-3Flag was used as a negative control. The solid and unfilled triangles point to the signals for intact Ebg1-GFP protein and the truncated Ebg1-GFP protein, respectively. d Co-localization of Ebg1-GFP and EF1a-mCherry in the apoplast of invasive hyphae of M. oryzae . An M. oryzae strain expressing Ebg1-GFP and EF1a-mCherry was used to inoculate rice sheath. The Ebg1-GFP/EF1a-mCherry image shows the overlay of GFP channel and mCherry channel. The merged image shows the overlay of GFP channel, mCherry channel, and the brightfield channel. Images were captured at 32 hpi on rice cultivar LTH. Scale bars = 20 μm. e EF1α inhibited Ebg1-triggered cell death in N. benthamiana . Cell death was observed in tobacco leaves infiltrated with Agrobacterium strains individually carrying EBG1 , EBG1 E378Q/E476Q , EBG1-N , or EBG1-C , but not in the leaves co-expressing EF1α with EBG 1, EBG1 E378Q/E476Q , EBG1-N , or EBG1-C . Pictures are representative tobacco leaves photographed at 7-day after agroinfiltration, and numbers indicate leaves with cell death versus total treated leaves. EV, empty vector. f Purified Ef1α protein partially blocks the Ebg1-induced ROS spiking in rice cultivar ZH11. Leaf disks of 4-week-old rice plants were incubated with 80 μg/ml Ebg1-6His with or without Ef1a-6His protein, and the luminol-based ROS burst was detected for 35 min constantly. Ef1a-6His protein alone and mock treatment were used as negative controls. RLU, relative light units. Error bars denote standard deviation, n = 8. g Δ ef1α mutants are significantly reduced in virulence on rice and barley. Rice and barley leaves were spray-inoculated with the conidial suspensions (3 × 10 4 spores/ml) of P131, Δ ef1α mutant, and complemented transformant Δ ef1α / EF1α , and photographed at 5 dpi. h Higher ratios of dark brown spots were formed on rice and barley leaves by Δ ef1α mutant than by P131. Numbers of typical lesions and dark brown spots on rice and barley leaves were counted per leaf. i Δ ef1α mutants fail to prevent ROS production. Rice sheath cells drop-inoculated with conidia suspensions (1 × 10 5 spores/ml) of P131, Δ ef1α , and Δ ef1α / EF1α strains were stained with DAB at 30 hpi, and the percentage of infection sites with DAB-stained cells was calculated. Scale bars = 20 μm. j Overexpression of EBG1 E378Q/E476Q in P131 driven by the EF1α promoter ( OEEBG1 E378Q E476Q ) resulted in reduced virulence on rice and barley leaves. Rice and barely leaves were spray-inoculated with conidial suspensions (5 × 10 4 spores/ml) of P131 and OEEBG1 E378Q/E476Q transformants. The inoculated leaves were photographed at 5 dpi. k Quantitative analysis of lesion formation on rice and barley leaves by P131 and OE EBG1 E378Q/E476Q transformants. Numbers of typical disease lesions and dark brown spots on rice and barley leaves were counted per leaf. l OE EBG1 E378Q/E476Q transformants induced ROS production. Rice sheath cells drop-inoculated with conidial suspensions (1 × 10 5 spores/ml) of P131 or OE EBG1 E378Q/E476Q transformants were stained with DAB at 30 hpi and the percentages of the DAB stained infection sites were calculated. Scale bars = 20 μm. For all the above statistics, error bars denote standard deviations from three biological replicates. ** and * indicate p < 0.01 and p < 0.05 significant differences compared with corresponding WT controls. One-way ANOVA with post-hoc Turkey tests were used in ( h ), ( i ), ( k ) and ( l ). Source data with statistic analysis are provided in a Source data file. Full size image A co-immunoprecipitation (Co-IP) assay showed that Ebg1 and EF1α could be immunoprecipitated by each other from filtrates of liquid CM cultures of a transgenic M. oryzae expressing EBG1-GFP and EF1α-3Flag (Fig. 5c ). We also collected apoplastic fluid of blast fungus-infected barley leaves and detected both Ebg1-GFP and EF1α-3Flag in the fluid (Supplementary Fig. 10c ), providing evidence that EF1α-3Flag protein can be secreted into the apoplast during M. oryzae infection. Further mass spectrometry analyses identified multiple peptides of Ebg1 and Ef1α in the filtrates of P131 liquid medium culture (Supplementary Data 1 ) and two peptides of Ef1α in the apoplastic fluid of barley leaves infected with P131 (Supplementary Data 2 ). Further, we generated transgenic M. oryzae co-expressing EBG1-GFP and EF1α-mCherry to check whether the two proteins are co-localized during infection. After inoculation of rice leaves with this transgenic M. oryzae strain, we observed that the fluorescence signals of Ebg1-GFP and EF1α-mCherry were partially co-localized in the apoplastic space of invasive hyphae (Fig. 5d ). These lines of evidence indicate that Ebg1 interacts and co-localized with EF1α in the apoplast during invasive growth of infection hyphae. To understand the biological relevance of the interaction between Ebg1 and EF1α, we transiently co-expressed EF1α and EBG1 or EF1a and EBG1 E378Q/E476Q in N. benthamiana . Surprisingly, cell death was not observed in tobacco leaves in these co-expression assays (Fig. 5e ), indicating that the presence of EF1α is sufficient to suppress the elicitor activity of Ebg1 and Ebg1 E378Q/E476Q . Immunoblotting confirmed that full-length Ebg1, and Ebg1 E378Q/E476Q were expressed as expected (Supplementary Fig. 10d ). Using a bimolecular fluorescence complementation (BiFc) assay, we also observed that Ebg1-nYFP interacted with cYFP-EF1α in the apoplast of tobacco leaf cells when they were transiently co-expressed (Supplementary Fig. 10e – g ). Furthermore, we verified that both the N and the C-terminal regions of Ebg1 could interact with the domain 2 and domain 3 of the EF1α protein in a Y2H assay and that EF1α also inhibited the elicitor activity of the Ebg1-N and Ebg1-C truncated proteins (Fig. 5b, e , Supplementary Fig. 10d ). To further investigate the effect of the presence of EF1α, we tested whether PAMP responses can be induced by purified Ebg1-6His protein in tobacco leaves that transiently expressed EF1α. The Ebg1-6His-induced MAPK activation was not detected in tobacco leaves pre-expressing EF1α (Supplementary Fig. 11a ). These data provide evidence that M. oryzae EF1α has the capacity to prevent Ebg1 from triggering plant immunity in tobacco leaves. In order to test whether Ef1α has an effect on Ebg1-induced rice immune responses, we purified Ef1α-GFP-6His protein from yeast strains (Supplementary Fig. 11b ) and tested its effects using purified Ebg1 proteins. Using anti-GFP beads, the Ef1α-GFP-6His protein could pull down Ebg1-GST protein in vitro (Supplementary Fig. 11c ). The purified Ef1α-GFP-6His protein did not inhibit the hydrolysis activity of Ebg1-6His on laminarin (Supplementary Fig. 11d ), but significantly suppressed Ebg1-induced ROS generation on rice leaves (Fig. 5f ). These data suggest that purified EF1 α protein prevents Ebg1 from triggering plant immunity in rice leaves. M. oryzae EF1 α is important for virulence The putative role of EF1α in suppressing the PAMP activity of Ebg1 suggested that EF1α may be important for virulence of M. oryzae . To test this idea, we generated Δ ef1α mutants in the M. oryzae P131 background (Supplementary Fig. 12a, b ). The Δ ef1α mutants grew normally on OTA plates (Supplementary Fig. 12c , d ), suggesting that EF1α is dispensable for normal mycelial growth and development of M. oryzae . However, the Δ ef1α mutants were notably reduced in their ability to cause blast disease in both rice and barley seedlings (Fig. 5g, h ). Furthermore, the Δ ef1α mutants also induced a ROS burst in rice leaf sheath cells (Fig. 5i ) and barley epidermal cells (Supplementary Fig. 12e ). EF1α is therefore important for virulence of M. oryzae . We reasoned that if Ebg1 interacts with EF1α to evade recognition as a PAMP, then this might require an excess of EF1α over Ebg1. To test this idea, we therefore generated an overexpression construct OE EBG1 E378Q/E476Q using the promoter of EF1α and transformed this into the wild-type M. oryzae strain P131. The resulting transformants showed consistently reduced virulence on rice and barley plants (Fig. 5j, k ) and induced a ROS burst in cells surrounding infection sites (Fig. 5l and Supplementary Fig. 12f ). Together, these data further suggest that Ebg1 is a PAMP that does not require its enzymatic activity to induce plant immunity and that M. oryzae normally suppresses its PAMP activity in a manner that requires EF1α. In addition, a pBLAST search suggested that orthologues of both Ebg1 and EF1α are widely distributed among fungi (Supplementary Fig. 1 and Supplementary Fig. 9 ). However, Ebg1 orthologues from different fungi are diversified in sequence while EF1α orthologues are highly conserved (Supplementary Figs. 1 , 9 , 13a, b ). Structural prediction indicates that Ebg1 from M. oryzae is highly similar to Ebg1 from Fusarium graminearum (Supplementary Fig. 13c ), suggesting that Ebg1 orthologues in different fungi may play similar roles. To test this idea, we performed Y2H assays, which showed that the Ebg1 and EF1α orthologues from F. graminearum could interact with each other, and that M. oryzae Ebg1 could also interact with F. graminearum EF1α, and vice versa (Supplementary Fig. 13d ). Furthermore, Ebg1 and EF1α orthologues from F. graminearum could largelly rescue the mutant phenotypes of Δ ebg1 and Δ ef1α mutants of M. oryzae , respectively (Supplementary Fig. 13e , f ). Together, these data suggest that the interaction between Ebg1 and EF1α in plant pathogenic fungi may be a conserved mechanism whereby fungal pathogens evade plant immunity and safeguard cell wall remodeling during infection. This study reports evidence that M. oryzae cell wall remodeling of β-1,3-glucan during plant infection involves at least two rounds of PTI and counter-PTI between the pathogen and host plant (Fig. 6 ). In the first round, plant cells recognize fungal β-1,3-glucans that are likely released by endo-β-1,3-glucanases during cell wall remodeling for invasive hyphal growth, consequently, initiating the first PTI to limit fungal colonization [14] , [43] (Fig. 3f, g ). To evade β-1,3-glucan-triggered plant immunity, M. oryzae secretes Ebg1, an exo-β-1,3-glucanase, to hydrolyze fungal-released β-1,3-glucans into glucose (Fig. 3d, e , Supplementary Fig. 5 ). As a response, the plant host perceives Ebg1 as a PAMP with an unknown receptor to activate the second PTI (Fig. 4b–e ). M. oryzae then appears to utilize an EF1α protein that interacts and co-localizes with Ebg1 to evade Ebg1-triggered PTI (Fig. 5b–f ). By evolving these two forms of counter-PTI mechanisms, M. oryzae is capable of protecting its cell wall from being recognized during infection without being detected by immune receptor(s) of host plants, thereby ensuring efficient colonization of plant tissues. Orthologues of both Ebg1 and EF1α are widely distributed among fungi (Supplementary Figs. 1 , 9 ). Our study further showed that Ebg1 and EF1α orthologues from F. graminearum could also interact with each other and could rescue the mutant phenotypes of Δ ebg1 and Δ ef1α mutants in M. oryzae , respectively (Supplementary Fig. 13 ). Therefore, the interaction between Ebg1 and EF1α may be a conserved mechanism of fungal pathogens to evade β-1,3-glucan-triggered host immunity during infection. Fig. 6: A working model for the potential mechanism by which Ebg1 and EF1α act to evade host plant immunity during invasive hyphal growth by M. oryzae . Fungal β-1,3-glucan fragments released by endo-β-1,3-glucanases at the fungal-plant interface can be perceived by a specific but unknown plant β-1,3-glucan receptor, and lead to PAMP-triggered plant immunity (PTI). M. oryzae expresses and secretes Ebg1 as an exo-β-1,3-glucanase hydrolyzing β-1,3-glucans into glucose to prevent the induction of PTI. Meanwhile, Ebg1 itself is a PAMP recognized by an unknown plant Ebg1 receptor to activate PTI. M. oryzae expresses an excess of EF1α protein, which is recruited by Ebg1, to evade the recognition of Ebg1, consequently preventing PTI. Full size image The M. oryzae Ebg1 identified in this study is an exo-β-1,3-glucanase of the GH17 family in fungi. Biochemically, Ebg1 is active on linear β-1,3-glucans and laminarin and produces only glucose as the end product (Fig. 3d, e ). Biologically, Ebg1 is important for M. oryzae to maintain cell wall integrity and cause blast disease (Fig. 1a–e ). Furthermore, Ebg1 triggers plant immune responses in a manner that is independent of its hydrolase activity (Fig. 4b, d ). These characteristics are distinct from that of CfGH17-1 in Cladosporium fulvum [44] , which is the sole β-1,3-glucanase of GH17 family characterized so far in filamentous fungal pathogens. CfGH17-1 is likely an endo-β-1,3-glucanase of the GH17 family that induces plant cell death depending on its enzymatic activity; however, it is not required for virulence by C. fulvum [44] . Ebg1 is also distinct from previously identified Scw4p, Scw10p, Scw11p and Bgl2p of S. cerevisiae [32] , [33] , [34] . Although these yeast proteins of the GH17 family function in cell wall remodeling, they are all endo-β-1,3-glucanases. Furthermore, Ebg1 also showed no similarity in amino acid sequence to previously reported exo-β-1,3-glucanases of the GH5 family, such as Exg1 in S. cerevisiae [45] , [46] , [47] and Candida albicans [48] , GLU1 in Pyrenophora tritici-repentis [49] , and Exo1 in Pythium insidiosum [50] , which are all important in cell wall remodeling. Interestingly, Exo1 is characterized as an intracellular immunoreactive protein triggering human cell antibody responses [51] , while M. oryzae Ebg1 is perceived by plant cells in the apoplast, suggesting that mammalian and plant host cells may have independently evolved mechanisms to recognize exo-β-1, 3-glucanase as a PAMP. Several previous reports have shown that GH proteins from filamentous plant pathogens can induce host immune responses without requiring enzymatic activity, including the GH11 member EIX from T. viride [52] , the GH12 member PsXEG1 from Phytophthora sojae [36] and the GH18 member MoChia1 from M. oryzae [26] . However, it remains largely unknown how fungal pathogens subvert perception of GH proteins by host plants. This study shows that Ebg1 can trigger plant immune responses, independent of its hydrolase activity (Fig. 4b, d ), and that EF1α can interact with both the N and C termini of Ebg1 and that this interaction prevents the triggering of cell death in transient co-expression assays in tobacco (Fig. 5b–e ). The interaction between Ebg1 and EF1α may therefore be the means by which the PAMP activity of Ebg1 is prevented during infection. Interestingly, EF1α has overall similarity to EF-Tu from Escherichia coli [53] , [54] and EF-Tu-a from Acidovorax avenae [55] (Supplementary Fig. 9 ), which are well-known bacterial PAMPs. E. coli EF-Tu contains the elf18 peptide with an acetyl-xKxKFxR motif crucial for inducing defense response in Brassicaceae species [53] , while the EFa50 from the Lys176 to Gly225 region of A. avenae EF-Tu-a could mount defense responses in rice [55] . However, EF1α lacks these motifs (Supplementary Fig. 14 ), consistent with its inability to induce cell death in tobacco plants (Fig. 5e ). The presence of EF1α appears to be necessary for M. oryzae to evade Ebg1-induced plant immune responses, but it remains unclear how these two proteins interact within the apoplast to evade Ebg1-triggered PTI. Further studies will therefore be required to identify a plant pattern recognition receptor that recognizes Ebg1 and to determine how this perception is prevented, or inhibited by the presence of EF1α. 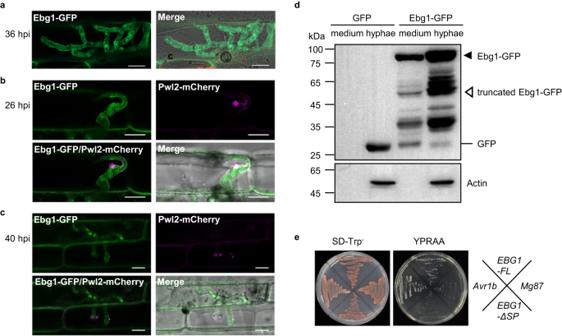Fig. 2: Ebg1 is a secreted protein. aSubcellular localization of Ebg1-GFP in the infection hyphae ofM. oryzae. The Ebg1-GFP fluorescence from the Δebg1/EBG1complemented transformants was distributed mainly around the cell wall and the tip of infection hyphae. Images were captured at 48 h post inoculation (hpi) on barley epidermal leaves. Scale bars = 20 μm.b,cLaser confocal micrographs ofM. oryzaestrain expressing Ebg1-GFP and Pwl2-mCherry. The Ebg1-GFP/Pwl2-mCherry image shows the overlay of the GFP channel and mCherry channel. A merged image shows the overlay of GFP channel, mCherry channel, and the brightfield channel. Images were captured at 26 hpi (b) and 40 hpi (c) on rice cultivar LTH. Scale bars = 10 μm.dThe Ebg1 protein was detected both in vegetative hyphae and cultured medium. A Δebg1/EBG1complemented transformant and a P131/GFPtransformant were cultured in liquid CM, and total proteins extracted from the mycelia and from the culture filtrates were immunoblotted with an anti-GFP antibody. Intact and truncated versions of Ebg1-GFP were labeled with a black solid triangle and an open triangle, respectively. Anti-actin antibody were used to confirm the protein samples of vegetative hyphae.eEbg1 has a functional signal peptide directing its secretion. TheEBG1full-length sequence (EBG1-FL) and signal peptide deleted sequence (EBG1-ΔSP) were constructed into the pSUC2 vector and transformed into yeast YTK12(SUC2-) for the invertase secretion test. The yeast transformants withEBG1-FLgrew well on the YPRAA medium containing raffinose and antimycin A, whereasEBG1-ΔSPfailed to grow on the same medium. Yeast strains withAvr1bandMg87were used as positive and negative controls, respectively. Strains and culture conditions M. oryzae P131 [31] , [56] was used as a wild-type strain to generate all mutants in this study (Supplementary Table 2 ). All M. oryzae wild-type strain and mutants were propagated on oatmeal agar medium (OTA) plates. Cell wall integrity was tested on complete medium (CM) [57] with 200 μg/ml CR and 100 μg/ml CFW, whereas the sugar utilization was examined on a minimal medium with 1% (w/v) glucose, laminarin, cellulose or chitin. Conidia were prepared as previously reported [56] . For M. oryzae inoculation, rice ( Oryza sativa cv LTH or NBT) plants were grown at 28 °C for 2–4 weeks, barley ( Hordeum vulgare cv E9) plants were grown at 28 °C for 5–7 days. Tobacco ( Nicotiana benthamiana ) plants were grown at 25 °C for 4 weeks before agroinfiltration or PAMP treatment. 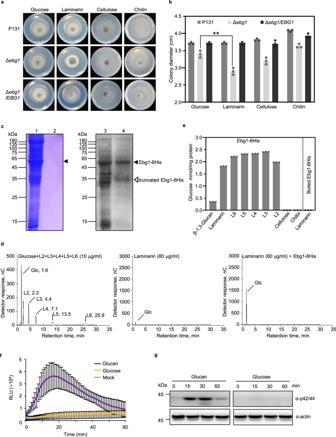Fig. 3:M. oryzaeEbg1 is an exo-β-1,3-glucanase. a,bThe growth of the Δebg1mutant on minimal medium with laminarin is significantly reduced compared to that on minimal medium with other polysaccharides as sole carbon sources. P131, Δebg1mutant, and Δebg1/EBG1were cultured on minimal medium supplemented with 1% (w/v) glucose, laminarin, cellulose, or chitin at 28 °C for 5 days, photographed (a) and measured for colony diameter (b). Laminarin, water-soluble β-1,3-linked glucans with occasional β-1,6-linked branches; Cellulose, β-1,4-linked glucans; Chitin, β-1,4-linked N-acetylglucosamine polymers. Error bars denote standard deviations from three biological replicates. **p< 0.01 using Student’sttest. Source data with statistic analysis are provided in a Source Data file.cPurification of Ebg1-6His protein from the CM culture filtrates ofM. oryzae. The crude proteins from liquid CM culture filtrates of anEBG1-6Hisstrain were purified with ion-exchange chromatography and polyhistidine binding resin before subjected to SDS–PAGE analysis with CBB staining (left panel) and immunoblot analysis using the anti-His antibody (right panel). Lanes 1 and 3: 10 μg of crude proteins; lanes 2 and 4: 0.5 μg and 0.25 μg of purified Ebg1-6His protein. The black solid triangles indicate the correct size for intact Ebg1-6His protein at around 55 kDa, and the open triangle indicates the truncated protein.dPurified Ebg1-6His protein hydrolyzed laminarins into glucose. Left panel: laminarioligosaccharides with different lengths (L2–L6) and glucose were loaded on HPLC as standard substances. Middle panel: untreated laminarin were loaded as blank control, and glucose was barely detected. Right panel: laminarin treated with purified Ebg1-6His protein were loaded for HPLC analysis and only glucose was detected from the reaction. Glc, glucose; L2, Laminaribiose; L3, Laminaritriose; L4, Laminaritetraose; L5, Laminaripentaose; L6, Laminarihexaose.ePurified Ebg1-6His protein hydrolyzed β-1,3-glucan, laminarin, and laminarioligosaccharides, but neither cellulose nor chitin. The hydrolytic activities of Ebg1-6His on different polysaccharides or oligosaccharides were assayed by detecting the amount of released glucose. Boiled Ebg1-6His protein lost its hydrolytic activity on laminarin. Error bars denote standard deviation.fROS burst was triggered by β-1,3-glucan but not glucose in rice. Leaf disks of 4-week-old rice plants were incubated with 20 μg/ml β-1,3-glucan or glucose, and the luminol-based ROS burst was detected for 60 min constantly. RLU, relative light units. Error bars denote standard deviation,n= 8.gMAPK activation was triggered in rice leaves by β-1,3-glucan but not glucose. Two-week-old rice seedlings were incubated with 40 μg/ml β-1,3-glucan or glucose for indicated time. Activated MAPKs were detected by immunoblotting with the phospho-p42/44 MAPK antibody. The anti-actin blot was used as a loading control. The experiment was repeated three times with similar results. Gene knockout and complementation EBG1 and EF1α knockout mutants were generated as reported [56] with the primers listed in Supplementary Table 3 . Protoplasts were isolated and transformed by the PEG/CaCl 2 method [58] . The mutants were first screened by PCR to detect flanking regions of hygromycin marker and then confirmed by Southern blot analysis. Probes used for Southern blot were labeled with the DIG High Prime DNA Labeling and Detection Starter Kit II (Roche). For complementation, the full-length EBG1 gene or EF1α containing a 1.5 kb native promoter fragment were amplified and cloned into pGTN [59] , and the resulting constructs were transformed into protoplasts of corresponding mutants. At least 15 neomycin-resistant complemented transformants for Δ ebg1/EBG1 or Δ ef1α/EF1α were picked up for functional tests, and the data from one complemented strain each were presented. The EBG1 E378Q/E476Q mutation was generated using PCR-based mutagenesis with the Q5 Site-Directed Mutagenesis Kit (NEB), and EF1a promoter was used as the overexpression promoter to drive EBG 1 E378Q/E476Q gene expression for functional tests. Virulence test and infection process observation To measure the virulence of M. oryzae strains, conidial suspensions at a concentration of 5 × 10 4 conidia/ml in 0.025% Tween 20 were sprayed on rice or barley leaves. The inoculated leaves were incubated in a moist, dark chamber at 28 °C for 30 h and then under regular illumination [56] . Disease lesions were scored and photographed at 5 day post-inoculation (dpi). 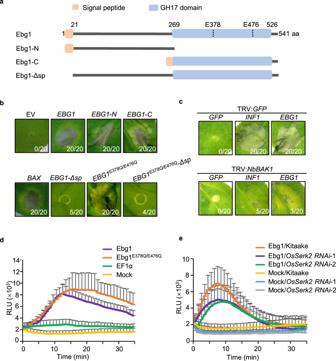Fig. 4: Ebg1 elicits tobacco cell death and activates rice immune responses. aSchematic diagram ofM. oryzaeEbg1 protein. The signal peptide is indicated in orange, and the GH17 hydrolase domain is indicated in blue. Ebg1, Full-length protein; Ebg1-N, the N-terminal half of Ebg1 (1-267aa); Ebg1-C, the signal peptide linked with the C-terminal half of Ebg1 (1-21aa fused to 268-541aa). Ebg1-Δsp, Ebg1 protein without the signal peptide.bEbg1 induced cell death inN. benthamiana. Tobacco leaves infiltrated withAgrobacteriumstrains carryingBAX,EBG1,EBG1-N,EBG1-C,EBG1-Δsp,EBG1E378Q/E476Q, andEBG1E378Q/E476Q-Δspwere photographed at 5-day post infiltration (dpi) and stained with trypan blue. The numbers indicate leaves with cell death versus total treated leaves. EV, empty vector was used as a negative control, and BAX was used as a positive control.cCell death triggered by Ebg1 inN. benthamianarequiresNbBAK1. Tobacco plants were subjected to VIGS by inoculation with TRV:GFPor TRV:NbBAK1. Three weeks after VIGS treatment,GFP,INF1, andEBG1were transiently expressed in the gene-silenced leaves and then leaves were photographed at 7 dpi. The numbers indicate leaves with cell death versus total treated leaves.dPurified Ebg1 protein induced ROS spiking in rice cultivar ZH11. Leaf disks of 4-week-old rice plants were incubated with 80 μg/ml Ebg1-6His or Ebg1E378Q/E476Q-6His, and the luminol-based ROS burst was detected for 35 min constantly. Ef1a-6His protein and mock treatment were used as negative controls. RLU, relative light units. Error bars denote standard deviation,n= 8.ePurified Ebg1 protein induced ROS generation in rice cultivar Kitaake and reduced ROS level in twoOsSerk2RNAi lines. Leaf disks of 4-week-old rice plants were incubated with 80 μg/ml Ebg1-6His, and the luminol-based ROS burst was detected for 35 min constantly. Mock treatment was used as the negative control. RLU, relative light units. Error bars denote standard deviation,n= 6. To investigate the infection process of M. oryzae strains, 3-week-old rice sheaths were injected with conidial suspensions of 1 × 10 5 conidia/ml in 0.025% Tween 20 and incubated in a moist, dark chamber at 28 °C. Microscopy observations were performed at 18, 24, 30, 36 h post-inoculation (hpi) under a Nikon 90i microscope. DAB staining and exogenous DPI and Ebg1 treatments Host-derived ROS was detected by staining rice sheaths with 3,3’-diaminobenzidine (DAB, Sigma-Aldrich). Rice sheaths or barley leaves inoculated with M. oryzae at 30 hpi, were immersed in 1 mg/ml DAB solution (pH 3.8) for 8 h and then de-stained overnight with the clearing solution (ethanol: acetic acid = 94: 4, v/v) before microscopic observation [60] . For assessing invasive growth of M. oryzae and ROS accumulation in rice sheath or barley leaves by the treatment of 0.5 μM diphenyleneiodonium (DPI) [59] or Ebg1-His, drop inoculation of M. oryzae conidial suspension was used, and DPI and Ebg1-His were added on the drop inoculation site at 12 hpi and in the conidial suspension, respectively. Subcellular localization of Ebg1 and co-localization of Ebg1 with EF1α A complemented strain Δ ebg1 / EBG1 expressing Ebg1-GFP was used to determine the subcellular localization of Ebg1, and a strain expressing Ebg1-GFP and Pwl2-mCherry was used to observe the localization of Ebg1 and Pwl2. A Nikon A1 laser scanning confocal microscope was used to observe the fluorescence distribution in vegetative hyphae cultured in liquid CM, conidia (0 h), conidial germ tubes (2 h), appressoria (24 h) on hydrophobic slides, and invasive hyphae of infected rice sheath cells at 20 and 40 hpi. To construct plasmid EF1α-mCherry with its native promoter for observing its co-localization with Ebg1, the EF1a coding sequence with native promoter was amplified using primers 3641-Pro-F and 3641-mCh-R and M. oryzae genomic DNA as template, and mCherry was amplified with primers mCh-Hind-F and mCh-Kpn-R. The resulting fragments were inserted into the SacII and KpnI digested site in pCB1532 by In-Fusion cloning. The plasmid EF1α-mCherry was then transformed into an M. oryzae strain expressing Ebg1-GFP. Positive transformants were selected by sulfonylurea resistance. Laser confocal microscopy was carried out to check the fluorescence of the transformants using a Leica SP8 laser confocal microscope. Yeast invertase secretion assay The yeast signal sequence trap vector pSUC2T7M13ORI (pSUC2) [61] , which carries a truncated invertase gene lacking signal peptide (SP), was used in this assay. The full-length EBG1 sequence ( EBG1-FL ) and SP-deleted coding sequences ( EBG1-∆ SP) were independently cloned into pSUC2 (Supplementary Table 3 ). The pSUC2-derived plasmids (0.5 µg) were transformed into the invertase-deficient yeast strain YTK12 (SUC2-) using the PEG/LiAc transformation method. Transformants were selected on yeast minimal tryptophan dropout medium (CMD-W medium, 0.67% yeast N base without amino acids, 0.075% tryptophan dropout supplement, 2% sucrose, 0.1% glucose, and 2% agar). Yeast colonies were then plated onto YPRAA plates (1% yeast extract, 2% peptone, 2% raffinose, and antimycin A at 2 µg/l) to detect the invertase secretion, Avr1b and Mg87 were used as the positive and negative controls, respectively. Purification of Ebg1 or Ebg1 E378Q/E476Q protein from M. oryzae liquid medium For protein purification, the coding sequence for six contiguous histidine residues was fused in-frame after the C-termial sequence of EBG1 or EBG1 E378Q/E476Q gene (Supplementary Table 3 ). The PCR product was ligated into the pRTN expression vector, and the resulting construct pRTN- EBG1 - 6His transformed into a Δ ebg1 mutant. A neomycin-resistant complemented transformant was used for protein expression and purification, which was cultured in liquid culture medium with 0.6% yeast extract, 0.3% casein enzymatic hydrolysate, 0.3% casein acids hydrolysate, and 1% sucrose at 28 °C, 160 rpm for 36 h. The culture was first filtrated with cheesecloth, and the filtrates concentrated by ultrafiltration (Vivaflow 50; Sartorius Stedim Biotech, Aubagne, France and Amicon Ultra-15; Millipore, Billerica, USA. 30 kDa) and equilibrated with 20 mM PBS buffer (pH 8.0) containing 150 mM NaCl [62] , [63] . Then, crude proteins were further purified with ion-exchange chromatography (IEC) and polyhistidine binding resin (TALON metal affinity resin; Clontech, CA, USA) with the PBS buffer. The resin was sequentially washed with 80 mM imidazole solution buffer containing 20 mM PBS (pH 8.0) and 150 mM NaCl. Finally, bound Ebg1-6His protein was eluted with a 300 mM imidazole solution buffer containing 20 mM PBS (pH 8.0) and 150 mM NaCl. The eluate was concentrated and equilibrated with 20 mM PBS buffer (pH 8.0) containing 150 mM NaCl by ultrafiltration (Amicon Ultra-4; Millipore, Billerica, USA. 30 kDa). The crude and purified Ebg1-6His proteins were subjected to SDS–PAGE followed by CBB staining and immunoblot analysis using an anti-His antibody [63] . Protein concentration was determined using a NanoDrop (NanoDrop One) or using a Bradford protein assay kit (Thermo-Fisher Scientific) with BSA (Sigma-Aldrich) as a standard. High-performance liquid chromatography (HPLC) analysis A Dionex ICS3000 system equipped with a pump, and pulsed amperometric detector, an automated sampler with a 25 μl injection loop, and a chromeleon chromatography management system (Dionex, Sunnyvale, CA) was used for sugar identification and quantification. The analytical CarboPac PA10 pellicular anion-exchange resin column (250 × 4 mm) preceded by a CarboPac PA10 guard column (50 × 4 mm) was used for sugar separation. The glucose was eluted with 25 mM NaOH at a flow rate of 1.0 ml/min, and then oligosaccharides were eluted with 150 mM NaOH. The mobile phase was prepared by diluting carbonate-free HPLC grade 50% (w/w) stock solution in distilled water, filtered with a 0.45 μm membrane, and degassed with compressed nitrogen gas for 30 min before loaded. Glucose mixed with laminarioligosaccharides (10 μg/ml each) (Laminarihexaose, L6; Laminaripentaose, L5; Laminaritetraose, L4; Laminaritriose, L3; Laminaribiose, L2 all from Megazyme) were used as standard substances. Untreated laminarin (80 μg/ml) (Sigma-Aldrich, L9634) was loaded as a blank control. A reaction mixture (100 μl) containing 0.2% laminarin or laminarioligosaccharides and 1.5 μg purified Ebg1-6His protein in 100 mM sodium phosphate (pH 5.0) was incubated at 50 °C for 2 h before loaded in HPLC machine. And a 15 μl aliquot of the end product was diluted with 485 μl of distilled water before ion chromatography (IC) injection. Enzymatic activity assay To assay the enzymatic activity of Ebg1, a 100 μl reaction mixtures containing 0.2% polysaccharides in 100 mM sodium phosphate buffer (pH 5.0) were incubated with 1.5 μg purified Ebg1-6His at 50 °C for 2 h. The glycosyl hydrolase activity of Ebg1 was calculated by the amount of released glucose using a glucose oxidase assay kit (Megazyme) [63] . A 50 μl aliquot of centrifuged supernatant was mixed with 50 μl glucose oxidase standard (GOS) and 200 μl POD overnight in a 96-well bottom clear plate (Costa). Then the absorbance value was measured at 510 nm by a microplate reader (SpectraMax i3x). The gradient glucose standards (50 μl) were used to draw the standard curve. Carbohydrates tested as substrates in this assay were β-1,3-glucan (Sigma-Aldrich, 89862), laminarin (Sigma-Aldrich, L9634), laminarin oligosaccharides (L2-L6) (Megazyme), cellulose (Sigma-Aldrich, S3504), and chitin from shrimp shells (Sigma-Aldrich, C9752). The optimal pH of Ebg1 was evaluated by equilibrating the reaction mixtures with 100 mM sodium acetate (pH 3.5–5.0), sodium phosphate (pH 5.0–7.5), Tris–HCl (pH 7.0–9.0), or sodium phosphate buffer (pH 9.0–12.0) for 12 h at 50 °C [62] . The optimal temperature for Ebg1 was examined by incubating reaction mixtures in 100 mM sodium phosphate (pH 5.0) for 12 h at 4, 10, 20, 30, 40, 50, 60, or 70 °C [62] , [63] . Agrobacterium tumefaciens infiltration assay in N. benthamiana The CDS of EBG1 , EBG1-N , EBG1-C, EBG1 E378Q/E476Q , and EF1α were cloned into the binary vectors pGWB414-3HA or pJL12-3Flag utilizing a pENTR TM Directional TOPO Cloning kit (Invitrogen) and Gateway LR Clonase II enzyme mix (Invitrogen). Constructs were introduced into A. tumefaciens strain EHA105 for the agroinfiltration of N. benthamiana leaves, as previously reported [38] . PCR confirmed Agrobacterium strains were cultured in YEP liquid medium (1% peptone, 1% yeast extract, and 0.5% NaCl, w/v) with suitable antibiotics and re-suspended in infiltration buffer (10 mM MgCl 2 , 10 mM MES, pH 5.6, and 200 μM acetosyringone) to a final OD 600 of 0.5 for 4 h prior to infiltration [64] . Two days after agroinfiltration, the leaves were punched with a 4 mm-puncher, and then proteins transiently expressed were extracted from 7 leaf disks with 120 μl 2.5 × SDS loading buffer. The proteins were subjected to SDS–PAGE with immunoblot analysis using an anti-HA antibody (Sigma-Aldrich) or an anti-Flag antibody (Sigma-Aldrich, A8592). For cell death observation, N. benthamiana leaves were photographed 5 days post infiltration [36] . The A. tumefaciens strain GV3101 carrying the pGR107:2Flag:BAX recombinant construct was used as a positive control for cell death. For virus-induced gene silencing (VIGS) assays, pTRV1, pTRV2: GFP , pTRV2: PDS , or pTRV2: NbBAK1 plasmid constructs were introduced into A. tumefaciens strain GV3101. The pTRV2: GFP , pTRV2: PDS , or pTRV2: NbBAK1 agrobacteria were mixed with pTRV1 agrobacteria in a 1:1 ratio for co-infiltration. The cultures were infiltrated into the primary leaves of N. benthamiana plants at the four-leaf stage. The effectiveness of the VIGS assay was evaluated with pTRV2: PDS three weeks after infiltration. The silencing efficiency of BAK1 was checked by RT-qPCR analysis. GFP , INF1 , and EBG1 were transiently expressed in the gene-silenced leaves after evaluation, and then leaves were photographed 7 d later. ROS burst and MAPK activation assay The leaves of 4-week-old N. benthamiana leaves were punched with a 4 mm diameter puncher for the ROS burst and MAPK assays as described previously [39] . For rice immune responses, 4-week-old rice plants and 2-week-old rice seedlings were used for ROS burst and MAPK assays, respectively. The leaf disks were kept in water overnight before the assays. For ROS burst assay, β-1,3-glucan or glucose were loaded in a final concentration of 20 μg/ml, Ebg1-6His or Ebg1 E378Q/E476Q -6His proteins were used in a final concentration of 80 μg/ml. The ROS signals were measured in a microplate reader at 450 nm (Spectra Max i3x). For MAPK assay, the activated MAPKs were detected by immunoblotting with the phospho-p42/44 MAPK antibody (CST), and anti-actin antibody (Abclonal) was used as a loading control. Quantitative RT-PCR assay To detect the expression of EBG1 at different M. oryzae infection stages and vegetative growth, barely leaves inoculated with conidial suspensions (8 × 10 5 spores/ml) of P131 at 0, 18, 24, 36, and 42 hpi were collected and the vegetative hyphae of P131 grown in CM liquid for 24 h were collected for RNA extraction. To detect the expression of BAK1 in VIGS treated N. benthamiana leaves, tobacco leaves with TRV: GFP and TRV: NbBAK1 at 3 weeks after infiltration were collected for RNA extraction. Total RNA was extracted with the KK Fast Plant Total RNA Kit (Zoman Biotechnology, Beijing, China). The first cDNA was synthesized with the HiScript II 1 st Strand cDNA Synthesis Kit (Vazyme, Nanjing, China), and Real-Time PCR then performed using 2×RealStar Green Power Mixture with ROXII (GenStar, Beijing, China) using specific primers (Supplementary Table 3 ). The expression of EBG1 was normalized to that of M. oryzae Actin gene, and the expression of BAK1 was normalized to EF1α of N. benthamiana . The experiments were conducted with three biological replicates, and one representative result was shown. Yeast two-hybrid (Y2H) assay The coding sequence (CDS) of EBG1-∆SP was cloned into the bait vector pGBKT7 (Clontech) to screen Ebg1-interacting proteins from a cDNA library constructed from with M. oryzae infected rice leaf tissues at 18 and 24 hpi. For Y2H validation, the CDS of EBG1- ∆SP, EBG1 E378Q/E476Q -∆ SP, EBG1 truncated versions were cloned into pGBKT7, and the CDS of EF1α and EF1α truncated versions, MGG_08162 and MGG_02504 were cloned into pGADT7 (Clontech) (Supplementary Table 3 ). The resulting bait and prey constructs were confirmed by PCR and then introduced into yeast strain Y2H-Gold as instructed (Clontech, BD library construction & screening kit). 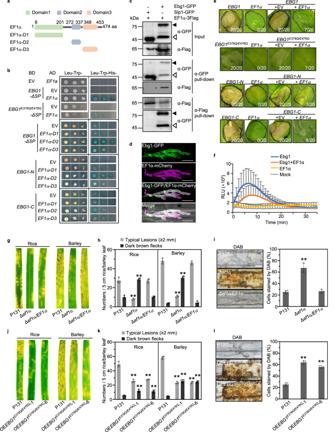Fig. 5:M. oryzaeEF1α interacts with Ebg1 and prevent plant immune responses triggered by Ebg1. aSchematic diagram ofM. oryzaeEF1α protein. Domain 1 with putative GTP binding activity, Domain 2 and Domain 3 with beta-barrel structure, are indicated in green, gray, and orange boxes, respectively. EF1α-D1, EF1α-D2, EF1α-D3 are truncations of EF1α protein with indicated domains.bThe yeast two-hybrid assays showing that EF1α-D2 and EF1α-D3, but not EF1α-D1 interact with Ebg1, Ebg1E378Q/E476Q, Ebg1-N, and Ebg1-C.cCo-immunoprecipitation assays showing that EF1α interacts with Ebg1 in the extracellular matrix ofM. oryzae. TheEBG1-GFPandEF1α-3Flagvectors were co-transformed intoM. oryzaeP131 for Co-immunoprecipitation assay. Total proteins from liquid CM culture filtrates of the transformant were subjected to GFP or Flag pull-down analysis. Total proteins or Co-IP elutions were detected by anti-GFP antibody or anti-Flag antibody. The P131 strain expressingSLP1-GFPandEF1α-3Flagwas used as a negative control. The solid and unfilled triangles point to the signals for intact Ebg1-GFP protein and the truncated Ebg1-GFP protein, respectively.dCo-localization of Ebg1-GFP and EF1a-mCherry in the apoplast of invasive hyphae ofM. oryzae. AnM. oryzaestrain expressing Ebg1-GFP and EF1a-mCherry was used to inoculate rice sheath. The Ebg1-GFP/EF1a-mCherry image shows the overlay of GFP channel and mCherry channel. The merged image shows the overlay of GFP channel, mCherry channel, and the brightfield channel. Images were captured at 32 hpi on rice cultivar LTH. Scale bars = 20 μm.eEF1αinhibited Ebg1-triggered cell death inN. benthamiana. Cell death was observed in tobacco leaves infiltrated withAgrobacteriumstrains individually carryingEBG1,EBG1E378Q/E476Q,EBG1-N, orEBG1-C, but not in the leaves co-expressingEF1αwithEBG1,EBG1E378Q/E476Q,EBG1-N, orEBG1-C. Pictures are representative tobacco leaves photographed at 7-day after agroinfiltration, and numbers indicate leaves with cell death versus total treated leaves. EV, empty vector.fPurified Ef1α protein partially blocks the Ebg1-induced ROS spiking in rice cultivar ZH11. Leaf disks of 4-week-old rice plants were incubated with 80 μg/ml Ebg1-6His with or without Ef1a-6His protein, and the luminol-based ROS burst was detected for 35 min constantly. Ef1a-6His protein alone and mock treatment were used as negative controls. RLU, relative light units. Error bars denote standard deviation,n= 8.gΔef1αmutants are significantly reduced in virulence on rice and barley. Rice and barley leaves were spray-inoculated with the conidial suspensions (3 × 104spores/ml) of P131, Δef1αmutant, and complemented transformant Δef1α/EF1α, and photographed at 5 dpi.hHigher ratios of dark brown spots were formed on rice and barley leaves by Δef1αmutant than by P131. Numbers of typical lesions and dark brown spots on rice and barley leaves were counted per leaf.iΔef1αmutants fail to prevent ROS production. Rice sheath cells drop-inoculated with conidia suspensions (1 × 105spores/ml) of P131, Δef1α, and Δef1α/EF1αstrains were stained with DAB at 30 hpi, and the percentage of infection sites with DAB-stained cells was calculated. Scale bars = 20 μm.jOverexpression ofEBG1E378Q/E476Qin P131 driven by theEF1αpromoter (OEEBG1E378Q E476Q) resulted in reduced virulence on rice and barley leaves. Rice and barely leaves were spray-inoculated with conidial suspensions (5 × 104spores/ml) of P131 andOEEBG1E378Q/E476Qtransformants. The inoculated leaves were photographed at 5 dpi.kQuantitative analysis of lesion formation on rice and barley leaves by P131 and OEEBG1E378Q/E476Qtransformants. Numbers of typical disease lesions and dark brown spots on rice and barley leaves were counted per leaf.lOEEBG1E378Q/E476Qtransformants induced ROS production. Rice sheath cells drop-inoculated with conidial suspensions (1 × 105spores/ml) of P131 or OEEBG1E378Q/E476Qtransformants were stained with DAB at 30 hpi and the percentages of the DAB stained infection sites were calculated. Scale bars = 20 μm. For all the above statistics, error bars denote standard deviations from three biological replicates. ** and * indicatep< 0.01 andp< 0.05 significant differences compared with corresponding WT controls. One-way ANOVA with post-hoc Turkey tests were used in (h), (i), (k) and (l). Source data with statistic analysis are provided in a Source data file. 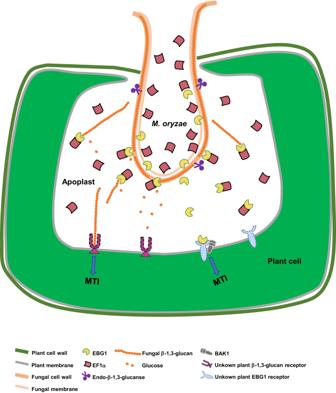Fig. 6: A working model for the potential mechanism by which Ebg1 and EF1α act to evade host plant immunity during invasive hyphal growth byM. oryzae. Fungal β-1,3-glucan fragments released by endo-β-1,3-glucanases at the fungal-plant interface can be perceived by a specific but unknown plant β-1,3-glucan receptor, and lead to PAMP-triggered plant immunity (PTI).M. oryzaeexpresses and secretes Ebg1 as an exo-β-1,3-glucanase hydrolyzing β-1,3-glucans into glucose to prevent the induction of PTI. Meanwhile, Ebg1 itself is a PAMP recognized by an unknown plant Ebg1 receptor to activate PTI.M. oryzaeexpresses an excess of EF1α protein, which is recruited by Ebg1, to evade the recognition of Ebg1, consequently preventing PTI. The yeast transformants grown on SD-Leu - Trp - medium were isolated and assayed for further growth on SD-Leu - Trp - His - medium. The expression of the Lac Z reporter gene was detected by X-α-gal according to the manufacturer’s instruction. Co-immunoprecipitation assay and western blotting To confirm the interactions of Ebg1 and EF1α in vivo, the genomic sequence of EBG1 was cloned into pGTN containing a GFP tag under its native promoter, while the genomic sequence of EF1α was cloned into pTH3Flag under its native promoter (Supplementary Table 3 ). The resulting constructs pGTN- EBG1 and pTH3Flag -EF1α were co-transformed into protoplasts of the wild-type strain P131. Transformants were screened on CM plates containing both neomycin (400 μg/ml, Ameresco) and hygromycin B (250 μg/ml, Roche). Total proteins from culture filtrates (CM) of the transformant expressing both Ebg1-GFP and EF1α-3Flag were incubated, respectively, with anti-GFP affinity resins (Chromotek, gta-20) and anti-Flag M2 affinity resins (Sigma-Aldrich, F2426). Proteins bound to resins were eluted after a series of washing steps following the manufacturer’s instruction. The total proteins and elution from resins were detected by western blotting. For western blotting detecting the presence of proteins, the following antibodes were used, anti-Actin (ABclonal, AC009, 1:2500), anti-Flag (Sigma, A8592, 1:5000), anti-HA (Sigma, H3663, 1:5000), anti-His (Abmart, 10E2, 1:5000), anti-p44/42 (Cell signaling, 9101, 1:2500), anti-GFP (Abclonal, AE012, 1:5000), anti-GST (EASYBIO, BE7012, 1:5000). Bioinformatic analyses M. oryzae GH17 family proteins or EF-Tu proteins were identified by a BLAST against NCBI database ( http://blast.ncbi.nlm.nih.gov/Blast.cgi ) with the amino-acid sequences of S. cerevisiae GH17 proteins (Scw4p, Scw10p, Scw11p, and Bgl2p) or M. oryzae EF1α. Orthologues of M. oryzae Ebg1 or EF1α were also obtained from NCBI ( http://blast.ncbi.nlm.nih.gov/Blast.cgi ). Sequences of other mentioned proteins in the article were searched following the NCBI accession numbers in related references. All accession numbers for the predicted protein sequences are provided in Supplementary Figs. 1 or 8 . Protein sequence identity and similarity were determined using EMBOSS Needle ( http://www.ebi.ac.uk/Tools/psa/ emboss_needle/ ). Sequence alignments were done using the MAFFT version7 ( https://mafft.cbrc.jp/alignment/server/ ) and BoxShade ( https://embnet.vital-it.ch/software/BOX_form.html ). Neighbor-joining phylogenetic trees were calculated in MEGA 6.0, using Bootstrap testing and 1,000 replications. Protein signal peptides were predicted by the SignalP ( http://www.cbs.dtu.dk/services/SignalP/ ). Protein domains were analyzed with SMART ( http://smart.embl-heidelberg.de/smart/set_mode.cgi?NORMAL=1 ). Protein structures of Ebg1 and FgEbg1 were predicted with Alphafold2 (Version 2.2.0, https://github.com/deepmind/alphafold ) [65] . Statistics and reproducibility For fungal growth assay, infection assay, DAB staining, and microscrope detection of fluorescence signals from Ebg1-GFP, experiments were repeated at least three times with similar results. For Southern blots and western blots, experiments were repeated at least two times with similar results, and one representative set of results or figures was shown. Image analyses were generated from Image J 1.54d. For all bar plots, data are represented as mean values +/−SD with datapoints shown as dots. Bar plots were drawn using GraphPad Prism 9. Statistical analyses were also performed in GraphPad Prism 9. Statistically significant differences were determined by one-way ANOVA and two-tailed Student’s t-test, and the exact p value was provided in the Source data file. Reporting summary Further information on research design is available in the Nature Portfolio Reporting Summary linked to this article.